Molecular architecture and the structural basis for anion interaction in prestin and SLC26 transporters Prestin (SLC26A5) is a member of the SLC26/SulP anion transporter family. Its unique quasi-piezoelectric mechanical activity generates fast cellular motility of cochlear outer hair cells, a key process underlying active amplification in the mammalian ear. Despite its established physiological role, it is essentially unknown how prestin can generate mechanical force, since structural information on SLC26/SulP proteins is lacking. Here we derive a structural model of prestin and related transporters by combining homology modelling, MD simulations and cysteine accessibility scanning. Prestin’s transmembrane core region is organized in a 7+7 inverted repeat architecture. The model suggests a central cavity as the substrate-binding site located midway of the anion permeation pathway, which is supported by experimental solute accessibility and mutational analysis. Anion binding to this site also controls the electromotile activity of prestin. The combined structural and functional data provide a framework for understanding electromotility and anion transport by SLC26 transporters. The high acuity of hearing in mammals requires an active mechanical process that boosts the sound-induced vibration in the inner ear [1] , [2] . ‘Cochlear amplification’ is provided by a highly specialized population of auditory sensory cells, the outer hair cells (OHCs). OHCs feature a unique high-frequency cellular motility driven by membrane potential changes [3] . This ‘electromotility’ is generated by prestin (SLC26A5) [4] , a membrane protein acting as an electromechanical transducer [5] . Prestin-mediated OHC electromotility underlies cochlear amplification, as shown by disruption of prestin function [6] , [7] . Dysfunction of prestin results in hearing loss in humans and in mouse models [8] , [9] . Prestin belongs to the mammalian SLC26 family of anion transporters that mediate translocation of various anions including chloride, bicarbonate, sulphate and oxalate [10] , [11] . SLC26 is part of the larger SulP family, including anion transporters in bacteria, plants, fungi and animals [12] . Biophysically, prestin most likely acts as an area motor by alternating between two structural conformations that occupy different cross-sectional areas within the membrane [13] , [14] . Joint conformational transitions of the tightly packed prestin motors in the plasma membrane of OHCs lead to macroscopic cellular length changes [5] , [13] . The distribution between both conformations is determined by the membrane potential, implying a mobile charged moiety acting as a molecular voltage sensor [15] that endows prestin with a motility-related charge movement or nonlinear capacitance (NLC) [16] . The molecular mechanism underlying electromotility may be related to the ion transport cycle in SLC26 transporters. Thus, non-mammalian prestin orthologues are electrogenic anion antiporters [17] , [18] and prestin-driven electromotility depends on anions at the intracellular side [19] , [20] , [21] , [22] . Despite a well-founded biophysical model for prestin’s electromechanical activity and a substantial body of structure–function studies [19] , [23] , [24] , [25] , the molecular mechanisms underlying piezoelectric activity and anion transport by SLC26 proteins have remained essentially unknown. Anion binding sites, permeation pathway and the protein domains undergoing the force-generating conformational rearrangements in electromotility await identification. So far, we identified two protein regions required for the generation of electromotility in mammalian prestin that also contain determinants for anion selectivity of non-mammalian SLC26A5, suggesting that they harbour core components of the molecular machinery for electromotility and anion transport [21] . However, further progress at the molecular level has been hampered by the lack of structural information for the entire SulP transporter family [12] , [26] . Here we present a structural model of mammalian prestin and the transport-competent orthologue from chicken (cPres), obtained by homology modelling using the crystal structure of the bacterial uracil transporter UraA as the template [27] . UraA is a member of the NCS2 protein family, which is related to SLC26/SulP proteins. Thus, sequence-based bioinformatic analyses indicate that the NCS2 and SulP families are the most closely related transporter families and assign sufficiently close homology to both groups [28] , [29] . The prestin homology structures were validated by molecular dynamics (MD) simulations and probed experimentally by extensive substituted cysteine accessibility scanning. We then used a mutational strategy to identify major parts of the translocation pathway and the central anion-binding site of SLC26 transporters. The findings highlight the same central site as the anion-binding site that controls electromechanical activity in prestin. The present results will provide the basis for deciphering the mechanistic details of electromechanical activity of prestin and thus of cochlear amplification. UraA as an appropriate template for homology modelling To identify a meaningful template for homology modelling, we screened the Transporter Classification Database (TCDB; www.tcdb.org [12] ) and the Pfam protein families database (pfam.sanger.ac.uk [30] ), which use different sequence-based methods to identify homology relationships between distantly related proteins. Both bioinformatic tools indicate that the nucleobase:cation-symporter-2 family (NCS2; SLC23; Xan_ur_permease in Pfam) is most closely related to SulP. Thus, Pfam uniquely relates the SulP family to the NCS2 family with an E -value 1.90 × 10 −6 , where E -values <10 −3 indicate close homology [30] . In full agreement, TCDB identifies NCS2 as most closely homologous to SulP with an s.d. score of 20.6, where a value of at least 11 s.d. is considered sufficient to establish homology [31] . In the TCDB database, SulP and NCS2 families cluster together in the same branch of the phylogenetic tree, indicating a common ancestor [29] . The evolutionary proximity of SLC26 SulP/SLC26 and NCS2 is further supported by two recent publications, an analysis of nearly 5,000 SLC transporter sequences [28] and a comprehensive comparison of human SLCs by sensitive profile–profile alignments [32] . The high-resolution crystal structure of one NCS2 member, the bacterial uracil transporter UraA, was reported recently [27] . Given that it is the available structure most closely related to SLC26A5, UraA is the most appropriate template for homology modelling of prestin. To further scrutinize a structural relationship between prestin and UraA, we submitted the prestin sequence to two homology detection algorithms, based on hidden Markov models (HMMs) and their profile analysis (HHpred server [33] ; Phyre2 (ref. 34) [34] ; see Methods). Profile HMMs make allowance for amino acid and insertion/deletion frequencies, and thus for the importance of each position for defining protein homologies. Pairwise comparison of profile HMMs is considered the currently most powerful and accurate method for detecting and aligning remotely related sequences [35] . Both HMM analyses yielded unambiguous results. Thus, HHpred server estimated the probability (that is, the degree of confidence) of homology between the entire transmembrane domains (TMD) of rPrestin and UraA as 100%. This remarkably high score is statistically supported by notable E -value (5E-38) and P -value (1.4E-35) scores. For comparison, the second meaningful hit returned by HHpred is a cyanobacterial Cl − /H + antiporter with poor scores (probability 7.9%, E -value 8.8E+2 and P -value 0.03). Similarly, the other HMM-based cutting edge protocol for homology recognition, Phyre2, returned the highest possible ‘confidence match value’ (100%) for the entire TMD of prestin versus UraA. Confidence values higher than 90% indicate that the central core of a derived structural homology model is accurate, that is, that deviation between derived homology model and the template three-dimensional (3D) structure is low (root mean squared deviation (r.m.s.d.) of 2–4 Å [34] ). In conclusion, four independent quantitative estimates (Pfam, TCDB, HHpred and Phyre2) converge to the same conclusion, indicating that UraA is the best available and a highly useful template for homology modelling of prestin. Modelling and MD simulations For structural analysis, we considered the electromechanically active mammalian prestin (rat prestin, rPres) and a transport competent, non-mammalian orthologue (chicken prestin, cPres [18] ). For homology modelling, we started from the sequence alignment of the core regions (TMD) of rPres (residues 74–502) and cPres (residues 73–506) to the UraA sequence derived from HHpred by pairwise comparison of profile HMMs [33] . Despite only modest sequence identity (10% and 12% for rPres and cPres, respectively), the HMM method produced a reliable alignment for the entire TMD ( Supplementary Fig. 1a ). Structures of the prestin TMD were modelled using the 3D crystal structure of UraA as the template [27] . The intracellular N and C termini were excluded from modelling, because the N terminus lacks a meaningful template and the C terminus, including the STAS domain whose structure is known [26] , has an uncertain orientation relative to the TMD. The r.m.s.d. between UraA and prestin homology models is in the range of 2–2.5 Å, major differences being due to the second and third extracellular loops that differ in length between the two families. To obtain validated and refined structural models, the initial homology models were submitted to 150 ns of MD simulations in a membrane system solvated by individual molecules of solvent (explicit solvation). This is an important a posteriori control of the energetic stability, as improperly modelled sequences (for example, choice of inappropriate template structure) are expected to deviate highly from the initial models in the course of the simulation, resulting in collapse and unfolding of secondary and tertiary structures. In the first 50 ns of simulation, rPres and cPres models moderately deviated from the starting models, reaching more favourable energetic states, reflecting differences between prestin and the template (UraA) sequence. As shown by asymptotic r.m.s.d. profiles ( Supplementary Fig. 1b,c ), structures reached equilibrium thereafter, indicating a stable and energetically favourable global fold. Despite local differences in the structures ( Supplementary Fig. 2 ), the final rPres and cPres MD models conserve the global fold and topology of UraA, thus energetically corraborating the validity of this transporter as the appropriate template. To select the final 3D prestin models used in further analyses, each MD trajectory was subjected to a cluster-based selection in the stable r.m.s.d. region using the SPICKER program [36] (see Methods). Main structural features The MD-derived structures of rPres and cPres conform to the characteristic fold of the UraA template structure: the prestin TMD comprises 14 TM segments organized into two structural repeats, TM1-7 and TM8-14, related by a pseudo two-fold inversion axis parallel to the membrane bilayer, yielding a 7+7 inverted repeat fold ( Figs 1a and 2 ). According to the UraA template, the TM segments are assembled into two major bundles ( Fig. 1b ) previously termed ‘core domain’ (consisting of TMs 1–4 and 8–12) and ‘gate domain’ (TMs 5–7 and 12–14) for UraA [27] . Consistent with secondary structure predictions, most TM segments exhibit a purely α-helical conformation, with the significant exception of two short antiparallel β-strands within TM3 and TM10 localized in the centre of the TMD. In UraA this unusual structural element plays a key role in coordinating the substrate, uracil. No disulphide bonds were detected, consistent with the conservation of function on replacement of all endogenous cysteines [37] , [38] . Two regions within the TMD of prestin (termed NLC1 and NLC2) are essential for electromotility and determine anion selectivity in a combinatorial manner [21] , [24] . This suggested a direct functional and possibly structural interaction of these regions, although both are far apart from each other in prestin’s primary structure ( Fig. 2 ). Strikingly, the rPres and cPres models now place NLC1 and NLC2 in intimate contact ( Fig. 1c ), thus conclusively explaining their functional interaction. 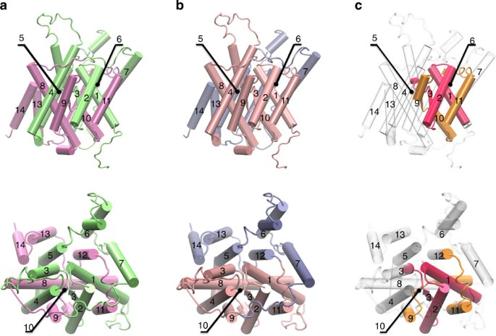Figure 1: Structural model of prestin derived by homology modelling and MD simulations. (a) Overall structure of the rPres TMD as derived from the MD simulation seen from the side (upper panel) and from the extracellular space (lower panel). Colours indicate the two inverted repeats (repeat TM1–TM7 in green, repeat TM8–TM14 in magenta). (b) Same prestin model, highlighting core (pink) and gate (blue-violet) domains, that were initially identified and defined for the UraA structure27. (c) Localization of the protein regions NLC1 (red) and NLC2 (orange) that have been implicated in the generation of electromotility and anion selectivity21. Although distant in the primary sequence (see alsoFig. 2) both regions interact closely, with their intertwined TMs building the core of the molecule. Specifically, these domains comprise the symmetry-related TMs 3 and 10 that are unusual in featuring central antiparallel β-sheets that contribute to substrate binding in UraA. Figure 1: Structural model of prestin derived by homology modelling and MD simulations. ( a ) Overall structure of the rPres TMD as derived from the MD simulation seen from the side (upper panel) and from the extracellular space (lower panel). Colours indicate the two inverted repeats (repeat TM1–TM7 in green, repeat TM8–TM14 in magenta). ( b ) Same prestin model, highlighting core (pink) and gate (blue-violet) domains, that were initially identified and defined for the UraA structure [27] . ( c ) Localization of the protein regions NLC1 (red) and NLC2 (orange) that have been implicated in the generation of electromotility and anion selectivity [21] . Although distant in the primary sequence (see also Fig. 2 ) both regions interact closely, with their intertwined TMs building the core of the molecule. Specifically, these domains comprise the symmetry-related TMs 3 and 10 that are unusual in featuring central antiparallel β-sheets that contribute to substrate binding in UraA. 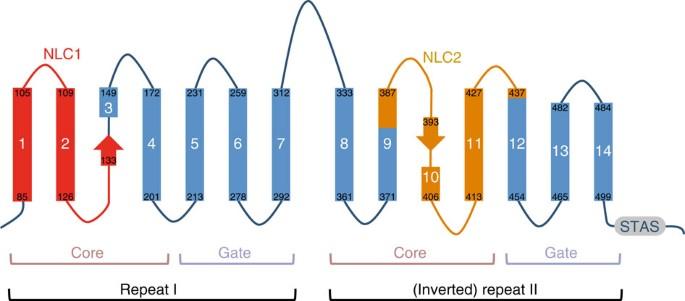Figure 2: Schematic representation of the topology and structural motifs of rPres. Cylinders represent helices, arrows represent the two β-strands β3 and β10 in TM3 and TM10. Protein regions NLC1 and NLC2 are highlighted in red and orange, respectively. Topological localization of repeats I and II and of core and gate domains are indicated. Each repeat can be superimposed onto the other (inverted) repeat by a 180° rotation around a symmetry axis parallel to the membrane. Black numbers refer to amino-acid positions in the rPres sequence. Cytoplasmic C and N termini not drawn to scale. Full size image Figure 2: Schematic representation of the topology and structural motifs of rPres. Cylinders represent helices, arrows represent the two β-strands β3 and β10 in TM3 and TM10. Protein regions NLC1 and NLC2 are highlighted in red and orange, respectively. Topological localization of repeats I and II and of core and gate domains are indicated. Each repeat can be superimposed onto the other (inverted) repeat by a 180° rotation around a symmetry axis parallel to the membrane. Black numbers refer to amino-acid positions in the rPres sequence. Cytoplasmic C and N termini not drawn to scale. Full size image Since the main structural features of rPres and cPres models are very similar ( Supplementary Fig. 2 ), below we focus on rPres. Experimental determination of topology confirms the models The membrane topology derived from homology modelling and MD simulations is unique and distinct from topologies proposed previously. Sequence-based 2D models suggested either 10 (ref. 39) [39] or 12 TM domains [19] , [24] , [40] , however, without unequivocal experimental support. To experimentally validate the structure, we thus determined prestin’s topology using a substituted cysteine accessibility method (SCAM) scan [41] . To this end we generated a prestin mutant devoid of cysteines (rPres ΔCys ) by replacing all endogenous cysteines by alanine. rPres ΔCys exhibited normal function, as indicated by wild-type-like electromotility-related charge movement, assayed as the bell-shaped NLC ( Supplementary Fig. 3 ). Subsequently, single cysteines were substituted into each predicted extra- and intracellular linker. Changes in NLC induced by application of thiol-reactive reagents to voltage-clamped cells were used as a functional assay for solvent accessibility of each cysteine-substituted position. The membrane-impermeable cysteine-reactive reagents (2-sulphonatoethyl)methane-thiosulphonate (MTSES) or [2-(trimethylammonium)ethyl]methane-thiosulphonate (MTSET) were applied either to the extracellular face of the membrane or to the cytoplasmic face via the patch pipette. Cysteine-free rPres ΔCys was entirely insensitive to application of either agent. In contrast, cysteine substitutions rendered prestin sensitive to MTSES or MTSET as indicated by changes in NLC properties. The observed changes were a shift of voltage dependence ( V 1/2 ), a change in NLC amplitude or the combined alteration of both parameters, as shown in Fig. 3a,b and Supplementary Fig. 4 . These changes indicated covalent modification and thus accessibility of the substituted site to either extra- or intracellular solutes and consequently location at the extra- or intracellular surface or within an aqueous pathway accessible from the respective side. For each of the predicted TM linkers, cysteine substitution of at least one position conferred reactivity to the thiol-reactive reagents, with the only exception of the very short linker between TM2 and TM3, which has a predicted intracellular localization. At this site, cysteine substitutions resulted in impaired membrane targeting or function, or mutants were insensitive to MTS reagents. Modification, and hence accessibility of each MTS-responsive position, was confined to either the intra- or the extracellular side. As summarized in Fig. 3c , cysteines at positions 104, 149, 236, 331, 389, 431 and 485 were readily modified by extracellular application of MTSES and/or MTSET. In contrast, positions 202, 276, 359, 408 and 465 were only accessible to MTSES and/or MTSET applied to the intracellular side whereas extracellular application had no effect on these mutants’ NLC. 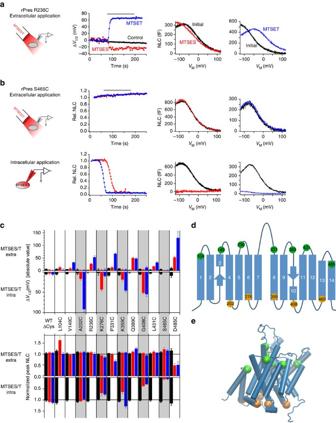Figure 3: Topology determination by substituted cysteine accessibility scanning. (a) rPresΔCys(R236C) as an example for an amino-acid position accessible from the extracellular side. NLC was measured in the whole-cell patch-clamp configuration while MTSES or MTSET (1 mM) were applied to the extracellular side via an application capillary (left panel). Changes inV1/2during the application (middle panel) indicate covalent modification of cysteine 236. Representative NLC traces before (black) and after application of MTSES (red) or MTSET (blue) are shown in the right panels. (b) rPresΔCys(S465C) as an example for an amino-acid position accessible from the intracellular side. Extracellular application of either MTSES or MTSET was totally ineffective (upper panels). Application of MTSES or MTSET (1 mM) to the intracellular side via the patch pipette (lower panels) abolished NLC with a time course consistent with diffusion of the reagents into the cytoplasm. (c) Summary of MTS modification results for all cysteine-substituted mutants obtained as inaandb. Data obtained with MTSES and MTSET are shown in red or blue, respectively. Black bars indicate control experiments without application of MTS reagents. The upper panel shows the absolute values ofV1/2shifts on application of MTSES or MTSET. For clarity, effects of extracellular application are plotted upwards and effects of intracellular application are plotted downwards. The lower panel shows relative (rel) changes in NLC amplitude on application of MTS reagents from the same set of experiments. As in the upper panel, amplitude changes in response to extracellular application are plotted upwards and effects of intracellular application are plotted downwards. Detailed data for each position are presented inSupplementary Fig. 4. Data are given as mean±s.e.m. withn≥5 experiments for each condition. (d,e) Schematic and structural representation of the results, showing the location of all examined amino-acid positions as predicted by the model. Positions accessible to MTS compounds from the extracellular side are coloured in green, those accessible from the intracellular side are coloured yellow. Figure 3: Topology determination by substituted cysteine accessibility scanning. ( a ) rPres ΔCys (R236C) as an example for an amino-acid position accessible from the extracellular side. NLC was measured in the whole-cell patch-clamp configuration while MTSES or MTSET (1 mM) were applied to the extracellular side via an application capillary (left panel). Changes in V 1/2 during the application (middle panel) indicate covalent modification of cysteine 236. Representative NLC traces before (black) and after application of MTSES (red) or MTSET (blue) are shown in the right panels. ( b ) rPres ΔCys (S465C) as an example for an amino-acid position accessible from the intracellular side. Extracellular application of either MTSES or MTSET was totally ineffective (upper panels). Application of MTSES or MTSET (1 mM) to the intracellular side via the patch pipette (lower panels) abolished NLC with a time course consistent with diffusion of the reagents into the cytoplasm. ( c ) Summary of MTS modification results for all cysteine-substituted mutants obtained as in a and b . Data obtained with MTSES and MTSET are shown in red or blue, respectively. Black bars indicate control experiments without application of MTS reagents. The upper panel shows the absolute values of V 1/2 shifts on application of MTSES or MTSET. For clarity, effects of extracellular application are plotted upwards and effects of intracellular application are plotted downwards. The lower panel shows relative (rel) changes in NLC amplitude on application of MTS reagents from the same set of experiments. As in the upper panel, amplitude changes in response to extracellular application are plotted upwards and effects of intracellular application are plotted downwards. Detailed data for each position are presented in Supplementary Fig. 4 . Data are given as mean±s.e.m. with n ≥5 experiments for each condition. ( d , e ) Schematic and structural representation of the results, showing the location of all examined amino-acid positions as predicted by the model. Positions accessible to MTS compounds from the extracellular side are coloured in green, those accessible from the intracellular side are coloured yellow. Full size image These SCAM results are consistent with solvent accessibility as derived from MD simulations ( Supplementary Fig. 5 ). Importantly, the pattern of accessibility is in full agreement with the predicted topology ( Fig. 3d,e ), corroborating the model and UraA as an appropriate template for modelling SLC26. Anion translocation pathway and substrate-binding site We next focused on the structural features that may be involved in anion transport in SLC26 transporters and in the control of electromotility by anions in mammalian prestin. The core of the TMD of the rPres and cPres models features a prominent cavity (around 500 Å 3 ), whose boundaries are formed by parts of TMs 1, 3 and 5 from the first repeat and by the symmetry-related TMs 8, 10 and 12, including the unusual antiparallel β-strands of TM3 and TM10 ( Fig. 4a ). This pocket structurally corresponds to the central substrate-binding site of UraA [27] . We hypothesized that in prestin this cavity also constitutes a central anion-binding site involved in electromotility and substrate transport. 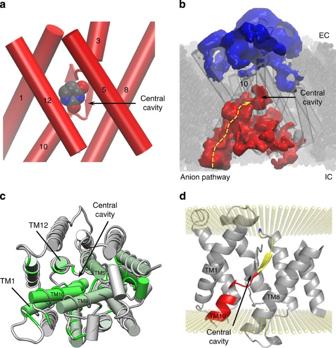Figure 4: The anion translocation pathway. (a) TM segments defining the central cavity. A uracil molecule is deliberately positioned corresponding to its location in the UraA crystal structure. (b) TMD cavities identified by analysis of solvent trajectories are shown in red (cavities accessible from cytoplasm, IC) and blue (accessible from extracellular solution, EC). The intracellular access pathway to the central cavity (yellow dashed line) was identified as a continuous solvated channel with a diameter compatible with passage of oxalate. (c) Intracellular view of the rPres model coloured according to TM segment distances from the anion pathway. Green helices are close to the pathway, distant helices are shown in grey. (d) Substituted cysteine accessibility confirms the model’s prediction of an inward-open anion access pathway for rPres. Shown is a lateral view onto the core domain summarizing the results of a SCAM scan along the entire TM10. Portions of the TM domain of rPres are not shown to enable view onto TM10. Experimental accessibility of TM10 residues to MTS reagents is indicated by colour code. Intra- and extracellularly accessible positions are highlighted in red and blue, respectively. Yellow positions were inaccessible from both sides. TM10 mutants at positions shown in grey were dysfunctional and could not be tested for accessibility. Original data are shown inSupplementary Fig. 6. Figure 4: The anion translocation pathway. ( a ) TM segments defining the central cavity. A uracil molecule is deliberately positioned corresponding to its location in the UraA crystal structure. ( b ) TMD cavities identified by analysis of solvent trajectories are shown in red (cavities accessible from cytoplasm, IC) and blue (accessible from extracellular solution, EC). The intracellular access pathway to the central cavity (yellow dashed line) was identified as a continuous solvated channel with a diameter compatible with passage of oxalate. ( c ) Intracellular view of the rPres model coloured according to TM segment distances from the anion pathway. Green helices are close to the pathway, distant helices are shown in grey. ( d ) Substituted cysteine accessibility confirms the model’s prediction of an inward-open anion access pathway for rPres. Shown is a lateral view onto the core domain summarizing the results of a SCAM scan along the entire TM10. Portions of the TM domain of rPres are not shown to enable view onto TM10. Experimental accessibility of TM10 residues to MTS reagents is indicated by colour code. Intra- and extracellularly accessible positions are highlighted in red and blue, respectively. Yellow positions were inaccessible from both sides. TM10 mutants at positions shown in grey were dysfunctional and could not be tested for accessibility. Original data are shown in Supplementary Fig. 6 . Full size image To identify the solute accessible pathways, we analysed the internal solvated areas by calculating the residence probability of explicit water molecules during the last 50 ns of the MD simulation with dxTuber [42] . The result of this analysis for rPres is reported in Fig. 4b ; essentially identical results were obtained for cPres. The central cavity is readily accessible from the intracellular space but occluded from the extracellular space by a constriction that precludes permeation from the exterior to the central cavity. Thus, the model captures rPres and cPres in an inward-open conformation, consistent with the inward orientation of the UraA template structure [27] . Using a dimensional filter based on the steric properties of oxalate, the largest substrate transported by non-mammalian prestins (see Methods), we identified a pathway connecting the cytoplasm with the central cavity that is consistent with the entry and accommodation of the known substrates of SLC26A5 (halides, sulphate, oxalate) [18] . It runs along TM10 and involves TM1, TM3, TM5, TM8 and TM12 ( Fig. 4b,c ). We propose that this pore constitutes the inner part of the anion translocation pathway. The occlusion towards the extracellular space indicates that in non-mammalian SLC26A5, full substrate translocation requires a major conformational change to provide an outward-facing conformation. Notably, the regions NLC1 and NLC2 comprising TM1, 3 and 10 ( Figs 1c and 2 ) make up a substantial part of the predicted anion transport pathway, which explains the strong impact of residues within these regions on anion selectivity and anion-dependent electromotility [21] . A SCAM scan along the entire TM10 provided experimental confirmation of the model results. As shown in Fig. 4d and Supplementary Fig. 6 , amino-acid positions predicted to contribute to the central cavity and its intracellular entrance S396–T406) were accessible to intracellular, but not extracellular MTS reagents. Towards the extracellular side, this stretch is preceded by residues (T390–C395) insensitive to application of MTSES reagents from either side of the membrane, indicating solute inaccessibility, which is consistent with a contribution to the permeation barrier between the main cavity and the extracellular side. Finally, Q389 at the extracellular tip of TM10 was selectively accessible to extracellular MTS reagents. We then probed residues predicted to contribute to the putative binding site by mutagenesis. In the UraA crystal structure, uracil is coordinated mainly by amino acids from TM3 and TM10, including G289 and E290 in TM10. Superposition of the UraA structure and the rPres model ( Fig. 5a ) shows that S398 in prestin corresponds to the important E290 in UraA. We focused on S398 and the neighbouring residue R399, located at the intracellular entrance of the central cavity ( Fig. 5a ). Both positions are entirely conserved in all vertebrate prestin orthologues ( Fig. 5b ) and largely throughout mammalian SLC26A paralogues, consistent with an important role in transport function. In analogy to chloride-binding sites in neurotransmitter transporters, serine side chains are obvious candidates for the coordination of anion substrates [43] , [44] . 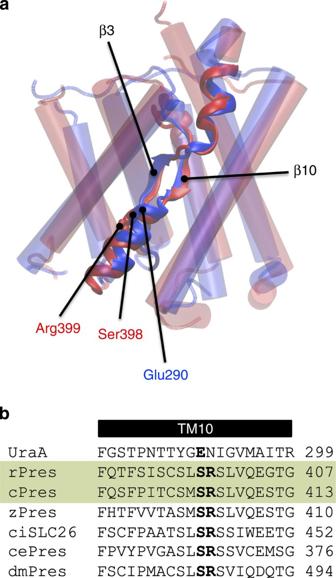Figure 5: Identification of a candidate central binding site. (a) Structural superposition of rPres (red) and UraA (blue). TM3 and TM10 are rendered in ribbon style, with antiparallel β-strands β3 and β10 as arrows. R399, S398 and Glu290 are highlighted, demonstrating the structural correspondence of Ser398 (rPres) to Glu290, which is involved in substrate binding in UraA. (b) Alignment of TM10 of UraA with various vertebrate prestins and invertebrate homologues (zPres=zebrafish prestin; ciSLC26, cePres and dmPres denote homologues fromCiona intestinalis(ciSLC26aα),Caenorhabditis elegans(Uniprot Acc. Q3LTR4) andDrosophila melanogaster(Q9VVM6), respectively). Sequence alignment with UraA is according to the structural superposition shown ina. Figure 5: Identification of a candidate central binding site. ( a ) Structural superposition of rPres (red) and UraA (blue). TM3 and TM10 are rendered in ribbon style, with antiparallel β-strands β3 and β10 as arrows. R399, S398 and Glu290 are highlighted, demonstrating the structural correspondence of Ser398 (rPres) to Glu290, which is involved in substrate binding in UraA. ( b ) Alignment of TM10 of UraA with various vertebrate prestins and invertebrate homologues (zPres=zebrafish prestin; ciSLC26, cePres and dmPres denote homologues from Ciona intestinalis (ciSLC26aα), Caenorhabditis elegans (Uniprot Acc. Q3LTR4) and Drosophila melanogaster (Q9VVM6), respectively). Sequence alignment with UraA is according to the structural superposition shown in a . Full size image Function was strongly impaired by mutation of R399 in rPres. Thus, the anion-dependent NLC was largely or fully abolished by mutation to cysteine, glutamine or glutamate, whereas substitution by lysine and serine preserved function, the latter yielding a strongly shifted voltage dependence ( Fig. 6a,b,e ). Mutation of S398 to cysteine produced a less dramatic phenotype, as NLC was preserved. However, careful examination showed that even the conservative exchange from serine to cysteine strongly affected the interaction with anions. We previously found that in mammalian prestin, binding of intracellular divalents reduces NLC, presumably by competing with chloride for an anion-binding site [21] . As shown in Fig. 6c,d , this inhibition by oxalate was strongly attenuated in the S398C mutant, indicating altered interaction with divalent anions. We used an additional measure to gauge the relevance of R399 in anion binding. Salicylate is a known inhibitor of prestin that competes with binding of intracellular chloride to prestin [19] , [45] , indicating a common or overlapping binding site. To examine the binding of salicylate, we probed the potency of inhibition by salicylate in a R399 mutant with preserved NLC (R399S). In rPres(R399S), inhibition of NLC by salicylate was abrogated and salicylate even enhanced NLC ( Fig. 6e,f ). Similarly, salicylate effects on NLC were also largely diminished in two other mutants that retained some NLC (R399T/C; Supplementary Fig. 7 ). These findings are consistent with the idea that R399 contributes to anion binding. 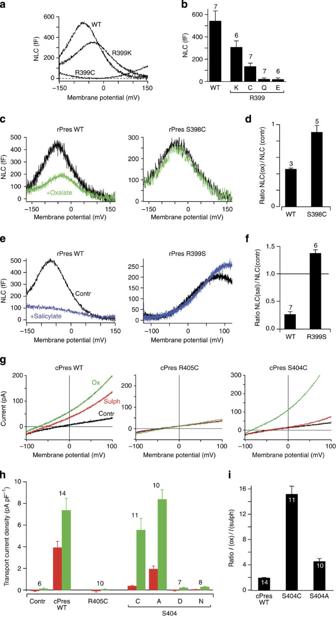Figure 6: Mutations in the central cavity affect NLC and anion transport. (a) Representative NLC recordings from the rPres mutants indicated. (b) Mean NLC amplitudes of rPres WT and R399 mutants. (c) Reduced oxalate (ox) sensitivity of NLC in the S398C mutant. Representative NLC traces from cells first recorded with standard pipette solutions (black) and subsequently repatched with a pipette solution containing additional 10 mM oxalate (green). (d) Mean fold change in NLC amplitude obtained as inc. (e) rPres R399S is insensitive to salicylate. Representative NLC recordings measured in control (contr) conditions (black) and from the same cells during application of 10 mM extracellular salicylate (blue). (f) Average fold changes in peak NLC amplitudes obtained from experiments as ine. (g) Representative transport currents from cPres and the mutants indicated in the absence of divalent substrates (black) and during subsequent application of extracellular 10 mM sulphate (red) or 10 mM oxalate (green). (h) Average transport currents of cPres-binding site mutant, normalized to cell size. Colour coding as ing. (i) Altered divalent selectivity of S404 mutants. Data were obtained from experiments as shown ing. The number of experiments (individual cells) is given in all bar graphs. Error bars indicate s.e.m. All described rPres and cPres mutants showed normal membrane localization, indicating intact folding and processing of the protein. Figure 6: Mutations in the central cavity affect NLC and anion transport. ( a ) Representative NLC recordings from the rPres mutants indicated. ( b ) Mean NLC amplitudes of rPres WT and R399 mutants. ( c ) Reduced oxalate (ox) sensitivity of NLC in the S398C mutant. Representative NLC traces from cells first recorded with standard pipette solutions (black) and subsequently repatched with a pipette solution containing additional 10 mM oxalate (green). ( d ) Mean fold change in NLC amplitude obtained as in c . ( e ) rPres R399S is insensitive to salicylate. Representative NLC recordings measured in control (contr) conditions (black) and from the same cells during application of 10 mM extracellular salicylate (blue). ( f ) Average fold changes in peak NLC amplitudes obtained from experiments as in e . ( g ) Representative transport currents from cPres and the mutants indicated in the absence of divalent substrates (black) and during subsequent application of extracellular 10 mM sulphate (red) or 10 mM oxalate (green). ( h ) Average transport currents of cPres-binding site mutant, normalized to cell size. Colour coding as in g . ( i ) Altered divalent selectivity of S404 mutants. Data were obtained from experiments as shown in g . The number of experiments (individual cells) is given in all bar graphs. Error bars indicate s.e.m. All described rPres and cPres mutants showed normal membrane localization, indicating intact folding and processing of the protein. Full size image Mutations in the homologous positions in the transport-competent cPres yielded equivalent results. Thus, anion transport by cPres was fully abolished by mutation to cysteine at position R405, homologous to R399 in rPres ( Fig. 6g,h ). Likewise, interaction with the divalent substrates was altered by mutation of S404 (S398 in rPres). In wild-type cPres, sulphate and oxalate are transported at similar rates (current ratio, 1.9±0.1) [18] . However, in cPres(S404C), sulphate transport was essentially abolished while oxalate transport was retained ( Fig. 6g–i ). Similarly, replacement of S404 by alanine altered anion selectivity. This altered anion interaction recapitulates the results obtained with the mammalian orthologue and supports an involvement of this position in the interaction of SLC26 with anions. Substitution with Asn (S404N) or the introduction of a negative charge at this site (S404D) entirely abolished transport activity, consistent with a more severe distortion of the substrate-binding site ( Fig. 6h ). Collectively, these functional observations on mutations in TM10 identify the central cavity as a major substrate-binding site of prestin, and most likely of SLC26 transporters in general. In particular, we conclude that the anion-binding site that controls electromotility and associated charge movement in mammalian prestin corresponds to the central binding site of the anion translocation pathway in SLC26 anion transporters. Conformational dynamics Occlusion of the substrate-binding site towards the extracellular solution suggests that substrate transport by transport-competent SLC26 proteins (for example, cPres) is mediated by alternate intra- and extracellular exposure of the central substrate-binding site (alternating access). To physically map prestin’s orientation, we probed the accessibility of a cysteine substituted into the substrate-binding pocket (rPres(S398C)/cPres(S404C); Fig. 7 ). In cPres, cysteine at position 404 readily reacted to MTS probes both from the extracellular and from the intracellular side. Extracellular application of MTSES, but not MTSET, rapidly inhibited divalent transport ( Fig. 7a,b ). The strong reactivity of extracellular MTSES prevented testing the intracellular efficacy of this probe, as cPres was already modified by extracellular MTSES leaking from the patch pipette while approaching the cell. However, intracellular MTSET introduced through the patch pipette abolished anion transport, revealing intracellular solvent accessibility of this site ( Fig. 7a,b ). The dual accessibility indicates a location of residue 404 at the centre of the protein, since it is inconsistent with a location at either the intra- or extracellular surface. We consider this as additional evidence for the validity of the prestin model structure and for the identification of the site as the central anion-binding site that is expected at a location midway across the membrane. Together, the dual modification of 404C demonstrates that the central anion-binding site is accessible to both intra- and extracellular solutes. Given that the experimental and computational structures of UraA and prestin, respectively, show occlusion of the binding site towards the extracellular space, we conclude that the dual accessibility of cPres results from the conformational dynamics of the transporter, with alternate exposure of the central binding site to the extra- and intracellular solutions during the transport cycle ( Fig. 7f ). 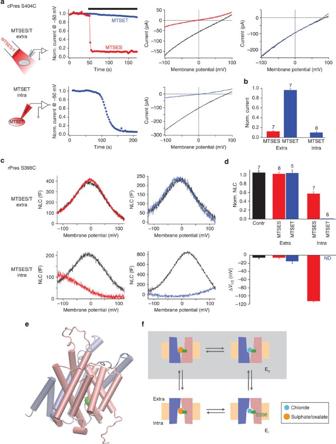Figure 7: Solvent accessibility of an amino acid in the proposed central binding site. (a) Upper panels, application of extracellular MTSES (0.1 mM; red) but not MTSET (1 mM; blue) to the extracellular side rapidly inhibits transport currents by cPres(S404C), indicating accessibility of this site. Lower panels, intracellular MTSET inhibits transport. Currents in the left panels are shown normalized to initial current (black). (b) Summary plot of remaining currents after application of MTS reagents obtained as ina. WT cPres was insensitive to both reagents (seeSupplementary Fig. 10). Error bars denote s.e.m. and the number of experiments is indicated above bars. (c) Representative NLC traces from rPresΔCys(S398C) obtained before (black) and after application of 1 mM MTSES (red) or MTSET (blue) from the extracellular (upper panels) or intracellular (lower panels) side. (d) Summary plot of NLC changes after application of MTS compounds obtained as inc. Upper panel shows fold changes of peak NLC. Lower panel presents MTS-induced changes ofV1/2. Error bars denote s.e.m. (e) Central location of residue S398 (green sphere) according to the structural model. Core (pink) and gate domains (blue-violet) indicated by colours. (f) Working model for alternating access transport mechanism consistent with the dual accessibility of position S404 in cPres. Alternate accessibility of the substrate-binding site may result from rotational movement between gate and core domains as hypothesized for UraA27. Shading of outward-facing conformation (Eo) symbolizes lack of extracellular accessibility of homologous position S398 in rPres, suggesting that outward-out conformation may not be reached. Figure 7: Solvent accessibility of an amino acid in the proposed central binding site. ( a ) Upper panels, application of extracellular MTSES (0.1 mM; red) but not MTSET (1 mM; blue) to the extracellular side rapidly inhibits transport currents by cPres(S404C), indicating accessibility of this site. Lower panels, intracellular MTSET inhibits transport. Currents in the left panels are shown normalized to initial current (black). ( b ) Summary plot of remaining currents after application of MTS reagents obtained as in a . WT cPres was insensitive to both reagents (see Supplementary Fig. 10 ). Error bars denote s.e.m. and the number of experiments is indicated above bars. ( c ) Representative NLC traces from rPres ΔCys (S398C) obtained before (black) and after application of 1 mM MTSES (red) or MTSET (blue) from the extracellular (upper panels) or intracellular (lower panels) side. ( d ) Summary plot of NLC changes after application of MTS compounds obtained as in c . Upper panel shows fold changes of peak NLC. Lower panel presents MTS-induced changes of V 1/2 . Error bars denote s.e.m. ( e ) Central location of residue S398 (green sphere) according to the structural model. Core (pink) and gate domains (blue-violet) indicated by colours. ( f ) Working model for alternating access transport mechanism consistent with the dual accessibility of position S404 in cPres. Alternate accessibility of the substrate-binding site may result from rotational movement between gate and core domains as hypothesized for UraA [27] . Shading of outward-facing conformation (E o ) symbolizes lack of extracellular accessibility of homologous position S398 in rPres, suggesting that outward-out conformation may not be reached. Full size image In rPres, cysteine substituted into the homologous position (S398C) was readily modified by intracellular MTSET or MTSES, as shown by a strong displacement of V 1/2 and decrease of NLC ( Fig. 7c,d ). In contrast to cPres, S398C was completely insensitive to both reagents applied to the extracellular face of the membrane ( Fig. 7c,d ), demonstrating accessibility from the cytoplasmic face only. Thus, both the structural model and the experimental accessibility are in agreement with the previous finding that mammalian prestin functionally interacts with intracellular anions only, but not with extracellular anions [19] , [21] , [45] . Hence experimental evidence now supports the previous notion that the conformational repertoire of mammalian prestin may be limited to inward-facing conformations [21] ( Fig. 7f ). Here we show for the first time a validated structural model of SLC26 transporters, focusing on the membrane motor prestin. The model is supported by several lines of evidence: phylogenetic analysis of the relation between SLC26/SulP and NCS2 transporters indicated UraA as the appropriate template for modelling; the 14 TM architecture was energetically stable by MD simulations and was supported experimentally by SCAM analyses. The results are further consistent with the extracellular localization of glycosylation sites N163 and N166 (ref. 46) [46] and with positions localized previously by introduced hemagglutinin tags [19] . While in principle the experimentally determined topology might also be consistent with a different structural fold, our further functional examination provides evidence supporting the presented 3D architecture. Thus, the model’s predictions for the central anion-binding site are consistent with the altered substrate binding observed when mutations were introduced at this site. Moreover, amino-acid 404 of cPres (corresponding to 398 in rPres) is solute accessible from both sides of the membrane, which physically maps this position to a central location within the permeation pathway. We consider this strong and independent support for one of the key features of our model, namely, the identity and location of the substrate translocation pathway. Finally, the 3D architecture of the model is strikingly consistent with previous findings, as it places two protein regions that interact functionally in determining electromotile activity and substrate specificity [21] in close and extensive contact, although these regions are located far apart in the primary sequence. Previously, a 12 TM topology model was derived experimentally for the bacterial SulP transporter, BicA [47] . Being largely similar to the current prestin model, the major difference is that the BicA model positioned the TM9/10 region (of the present prestin model) as an intracellular loop. Since the previous approach used truncated protein fused to a tandem enzymatic reporter construct [47] , it may easily lead to structural misfolding at the truncation/fusion region. In contrast, our approach is much less disruptive in introducing single point mutations, and included an intrinsic control for correct folding, since all mutants analysed were fully functional. Moreover, the present data unequivocally refute previously proposed topologies featuring either 10 or 12 TM-spanning domains [19] , [24] , [39] , [40] , [48] , because the 10 and 12 TM models place many residues opposite to the experimental SCAM results ( Supplementary Fig. 8a,b ). The prestin structure provides a rational for the specific role of two sequence motifs previously recognized for their conservation throughout the SulP/SLC26 family, the ‘SulP consensus signature’ (Prosite PS01130) and a motif first recognized by Saier et al. [49] (‘Saier motif’ [11] ). The conserved SulP and Saier motifs correspond to TM2 and TM9–10, respectively ( Supplementary Fig. 9 ), overlapping with the functionally defined regions NLC1/2 (ref. 21) [21] . Notably, symmetry-related TM2 and TM9 interact strongly ( Fig. 1 ), revealing a direct contact of both conserved motifs that has not been recognized before. Ohana et al. [50] recently suggested that a conserved glutamate within the Saier motif (E374 in rPres) is involved in anion permeation in SLC26 transporters. Their suggestion was based on a homology model of SLC26A6 using the Cl − /H + transporter ClC-ec1 as the template. While the SCAM analysis refutes the ClC-based model ( Supplementary Fig. 8c ), our model provides another explanation for conservation and functional importance of this residue: E374 interacts with highly conserved Y123 within the SulP motif (TM2). We hypothesize that these two conserved residues are important for the TM2–TM9 association. Structurally, both TM helices appear to provide a shell or scaffold for the non-helical (symmetry-related) immediately adjacent TMs 3 and 10, which constitute the centre of the core domain. Most SLC26s function as coupled anion antiporters [11] , [51] . Although the underlying mechanisms are largely unknown, the stoichiometric antiport is most easily explained by an alternating access mechanism, where a central binding site is alternately exposed to either side of the membrane. Binding of a substrate enables a major conformational change that results in exposure and substrate release to the opposite side. Subsequent binding of the counter-transported substrate allows for the reverse conformational switch, thus completing the antiport cycle ( Fig. 7f ). On the basis of the inward-open structure of UraA, the prestin model portrays SLC26A5 in an inward-facing conformation: it exhibits an intracellular access channel to a central binding site occluded from the extracellular space. Consistent with the structure, the inner cavity (S398/404C) of mammalian and non-mammalian prestin was accessible to thiol-reactive compounds from the intracellular space. The additional modification by extracellular MTSES in cPres indicates that in the transport-competent SLC26s, the same site also experiences exposure to the extracellular medium. Since the entire population of transporters was shut down by either intra- or extracellular MTS reagents, we conclude that the binding site rapidly switches between extra- and intracellular exposure, which provides direct evidence for alternate access. We note that simultaneous accessibility from both sides to large solutes such as the MTS compounds is unlikely, because this would imply a continuous and large-diameter permeation pathway allowing for uncoupled permeation of smaller anion substrates such as chloride, which is not observed [18] . Taken together, structure and experimental accessibility studies support alternate access as the mechanism of coupled anion transport in SLC26 transporters, as also found for various secondary transporters of the APC (amino acid-polyamine-organocation) superfamily that have been studied in much more detail [52] . SLC26 transporters generally appear to form dimers or tetramers [53] , [54] and in mammalian prestin, the subunits interact functionally [55] . Although the present structure does not provide information on oligomerization, the central location of binding site and anion pathway clearly show that each subunit must contain its own translocation pathway. The new structure may also provide insights into the molecular mechanism of electromotility of mammalian prestin. Electromotility and associated charge movement (NLC) are thought to involve a major voltage-driven conformational change [5] , [13] , [14] . Given the inward-to-outward transition during the transport cycle in cPres, it is tempting to speculate that this structural reorientation may also result in changes in the molecule’s overall dimensions, thereby generating the electromotile length changes. Thus, inward-open and outward-open conformations may occupy different areas in the plane of the plasma membrane. On the basis of a series of high-resolution crystal structures, a quite detailed picture of the structural mechanism of substrate transport has emerged for NSS transporters (neurotransmitter sodium symporters) that are more distantly related to SulP with the bacterial amino-acid transporter LeuT as the structural prototype [52] . Despite structural differences, the TCDB and Pfam databases and the most recent sequence-based bioinformatics analyses group SulP (and NCS2) transporters into the same APC superfamily that includes the NSS family [28] , [29] . LeuT features a 5+5 inverted repeat fold [56] and alternating access transport is thought to be mediated by the tilting movement of a bundle of TMs behaving as a rigid body [52] . Although the structural relation of the 7+7 fold to the 5+5 architecture of LeuT remains to be analysed, the fundamental similarity, that is, interdigitated inverted repeats, and the phylogenetic relation suggest a similar mechanism in SulP and NCS2 transporters. For UraA, a tilting motion of the gate domain relative to the core domain was suggested as the conformational switch that reorients the central substrate-binding site between intra- and extracellular side [27] . In fact, movement of a rigid TM bundle seems ideally suited to exert force against external load as observed in the collective electromotile behaviour of prestin populations. Whatever the precise mechanistic relation of electromotility and the molecular mechanics of anion transport may be, the structural model now clearly shows that the main determinants for electromotile activity make up the core of the transport pathway. Moreover, the model provides a structural rational for the well-established anion sensitivity of electromotility and associated charge movement/NLC [19] , [20] . Recent work suggested that binding of intracellular chloride precedes the major voltage-driven conformational change that generates charge movement and associated area change [21] , [22] . Several lines of evidence now indicate that the binding site fundamental for electromotility is identical to the central anion-binding site of the transport pathway. Structurally, the transporter’s binding site is fully conserved in mammalian prestin. Physical mapping with thiol-reactive probes showed that in mammalian prestin the central cavity is accessible for intracellular solutes only, recapitulating the exclusive influence of intracellular, but not extracellular, anions on prestin’s electromotile activity. Furthermore, mutations in the central binding site either abolished NLC or strongly affected the ability of oxalate and salicylate to compete with the chloride required to support electromotility/NLC. A number of obvious questions remain to be addressed. Arguably, the most interesting is the identification of the domains that move in response to a voltage change and thereby drive electromotility. The model also does not provide an immediate answer to the long-standing question of how charge movement (NLC) comes about. Mobile anion substrate [19] or charged protein domains [23] have been suggested as the mobile voltage sensor. Furthermore, what is the structural basis for the lost [18] , [21] or reduced [57] transport activity of mammalian prestin? In conclusion, the proposed structure of mammalian and non-mammalian prestins is strikingly consistent with a wealth of experimental data and should provide an important framework for addressing the unresolved mechanisms of electromotility and anion transport by SulP family transporters. Undoubtedly, experimental high-resolution crystal structures will be needed for detailed atomic level analysis of the anion transport cycle and its involvement in electromotility. Homology modelling To identify appropriate templates, the sequences of mammalian prestin and homologues were submitted to homology recognition algorithms based on HMM profile alignment techniques, considered most appropriate for detecting remote homologies [35] . In unbiased searches, both methods, HHpred (Homology detection & structure prediction by HMM-HMM comparison, http://toolkit.tuebingen.mpg.de/hhpred ) [33] and Phyre2 ( http://www.sbg.bio.ic.ac.uk/phyre2 (ref. 34 )), returned UraA as the best and the only reliable target, consistent with Pfam and TCDB databases. Metrics indicating the reliability of structural relation were unambiguous: HHpred returned ‘probability’ 100.0%, E -value 5E-38 and final HHpred Score 319.3; and Phyre2 yielded the highest possible confidence value (100%). We then used the structure of UraA (Protein Data Bank (PDB) code 3QE7) as the template for modelling the TMD region of the sequences of rat prestin (UniProt: Q9EPH0) and chicken prestin (UniProt: A0FKN5). Homology modelling was performed with the Homology Model tool implemented in the Molecular Operating Environment software suite (MOE, version 2010, www.chemcomp.com ). For the correct identification and positioning of the secondary structure elements, we started from the prestin-to-UraA alignment derived by the HHpred server. Hence, initially, backbone atom coordinates for transmembrane segments only were obtained from the relative coordinates of UraA. In case of residue identity, also side chain coordinates were copied. Subsequently, insertions and deletions were included and their backbone modelled. Loops were modelled on the basis of the structure of compatible fragments found in the PDB, and side chains were picked from a rotamer library by a deterministic procedure based on unary quadratic optimization to select optimal packing, according to methods implemented in MOE. In the final step, models were submitted to energy minimizations to reduce steric contacts (r.m.s. gradient, r.m.s.=0.5). In this way, 50 initial models based on the CHARMM27 force field [58] were generated, all sharing the same TMD topology but differing in local conformations. The quality of the models was evaluated by MOE protein geometry tools and scored according to the generalized Born/volume integral model [59] . The energetically most favourable model (for rPres and for cPres) was selected for analysis by MD. MD simulations Both homology models were submitted to 150 ns of MD simulation. Models were inserted into a 1-palmitoyl-2-oleoyl-sn-glycero-3-phosphocholine membrane bilayer extending 110 × 110 Å in the X–Y plane, solvated with roughly 5.6 × 10 4 water molecules (TIP3P water model) and 0.150 M NaCl, as described recently [60] . MD simulations were based on CHARMM27 force field and the particle-mesh Ewald's method for long-range electrostatic treatment (cutoff 9 Å and switchdist 7.5 Å). An initial equilibration was carried out by 3,000 steps of energy minimization followed by 20 ns of isothermal–isobaric ensemble (NPT mode, that is moles (N), pressure (P) and temperature (T) are conserved) MD simulation, in which the protein was kept constrained while the membrane and water were equilibrated. A further equilibration step of 10 ns was performed decreasing by a factor of 10 the harmonic constant applied to constrain the protein atoms. During both equilibration steps, the Langevin thermostat was applied to maintain 310 K, adjusting the kinetic energy of the particles with a Langevin damping equal to 0.1; the pressure was controlled by Berendsen barostat and set at 1 atm. In the production step, a simulation of 150 ns was carried out without constrain in the canonical ensemble (NVT mode, that is moles (N), volume (V) and temperature (T) are conserved) using Langevin thermostat set at 310 K. All simulations were carried out using ACEMD_25.80 software [61] , running on GeForce GTX480 Nvidia GPU. Cavities were identified analysing the last 50 ns of both solvent and protein trajectories with the dxTuber_0.25 tool [42] , using the default 0.1 and 0.3 minimum density values for protein and solvent, respectively. Analysis of the water accessibility was performed evaluating the frequency of contacts of each residue with water molecules on each frame extracted in the last 10 ns of the MD simulation. The frequency was then normalized to residues showing water contacts during the entire period analysed. The anion pathway was identified selecting cavities with a diameter larger than the oxalate sterimol size parameter ‘ L ’ [62] as a good descriptor of the molecular size. For each MD simulation the representative (final) model was selected using the SPICKER_2.0 tool [36] , which identifies the near-native models. Briefly, frames were grouped according to both structural similarity and potential energy, and the structure closest to the centroid of the most populated group was selected. Molecular biology cDNAs coding for SLC26A5 from Rattus norvegicus (rPres) and Gallus gallus (cPres) were cloned into pEGFP-N1 expression vector (Clontech Laboratories, Mountain View, CA, USA), yielding C-terminal green fluorescent protein fusion constructs described previously [18] , [21] . Point mutations were introduced using QuickChange Site-Directed Mutagenesis Kit (Agilent Technologies, Santa Clara, CA, USA). All constructs were verified by sequencing. Electrophysiology Plasmid DNA was transfected into Chinese hamster ovary cells using JetPEI transfection reagent (Polyplus, Illkirch, France). For electrophysiological experiments (24–48 h after transfection), cells with unequivocal membrane fluorescence were selected. Whole-cell patch-clamp recordings were carried out at room temperature (20–22 °C) with EPC10 amplifiers (Heka, Lambrecht, Germany) controlled by Patchmaster software (Heka). NLC recordings Patch pipettes were filled with an intracellular solution containing (in mM) 160 CsCl, 1 HEPES, 1 K 2 EGTA (pH 7.3 with CsOH). For experiments addressing competition between intracellular chloride and oxalate, intracellular chloride concentration was set to 10 mM. Here, pipette solution was either (in mM) 10 CsCl, 10 Na 2 -oxalate, 135 Na-aspartate, 1 K 2 EGTA, 1 HEPES or 10 CsCl, 150 Na-aspartate, 1 HEPES (pH 7.3 with NaOH). Extracellular solution was (in mM): 144 NaCl, 5.8 KCl, 1.3 CaCl 2 , 0.9 MgCl 2 , 10 HEPES, 0.7 Na 2 HPO 4 , 5.6 glucose (pH 7.4 with NaOH). Whole-cell membrane capacitance ( C M ) was recorded using the sine+DC software lock-in function of Patchmaster utilizing 2 kHz stimulus sinusoids. Voltage-dependent NLC was assessed by recording C M during voltage ramps as described [17] and plotted as a function of membrane potential ( V M ). Traces shown usually represent averages from 2 to 10 individual capacitance traces. NLC was quantified by fitting the derivative of a first-order Boltzmann function to the C M ( V M ) traces, where C lin is linear membrane capacitance, V M is membrane potential, Q max is maximum voltage-sensor charge moved through the membrane electric field, V 1/2 is voltage at half-maximal charge transfer and α is the slope factor of the voltage dependence. The amplitude of NLC was quantified as peak NLC, NLC max = C M ( V 1/2 )− C lin . Transport measurements Electrogenic anion transport was measured as the ionic transport current in response to command voltage ramps (−100 to +100 mV) as described previously [18] . Transport was elicited by addition of divalent transport substrates to either the intracellular or extracellular solution. For quantification of transport activity across different cells, average currents are given as current densities (pA/pF), obtained by normalizing to membrane capacitance, which is a measure of membrane area. For extracellular application of divalents, the extracellular solutions contained (in mM) 10 NaCl, 10 Na 2 -oxalate or 10 Na 2 SO 4 , 130 Na-gluconate, 2 Mg-gluconate, 10 Hepes (pH 7.4 with NaOH); extracellular solution for control (baseline currents) was 10 CsCl, 150 Na-gluconate, 2 Mg-gluconate 2 , 10 HEPES (pH 7.4 with NaOH). Pipette solution was (in mM) 160 CsCl, 1 HEPES, 1 K 2 EGTA (pH 7.3 with CsOH). In case of intracellular application, extracellular solution was as described for NLC recordings and pipette solution contained (in mM) 10 CsCl, 10 Na 2 -oxalate, 135 Na-aspartate (pH 7.3 with NaOH). An agarose bridge was used as the bath electrode whenever extracellular anions were exchanged. Cysteine modification Stock solutions (0.2 M) of MTSES or MTSET were prepared in dimethylsulphoxide (DMSO) and stored frozen at −20 °C until use. MTSES or MTSET were added to intracellular or extracellular solutions immediately before use. Final concentration of DMSO in intra- or extracellular solutions was 1% or less. Since MTS compound leaking from the patch pipette rapidly modified cysteine-substituted positions accessible from the extracellular side before establishing whole-cell configuration, these positions could not be tested for MTS effects from the intracellular side. To identify cysteine-reactive residues for experimental determination of topology, several residues within each predicted TM–TM linker were substituted by cysteine. Mutants were screened for membrane localization and NLC to control for correct protein folding and function. Further analysis focused on one cysteine substitution per TM–TM linker with robust NLC and sensitivity to MTS reagents. Data are given as mean±s.e.m. How to cite this article: Gorbunov, D. et al. Molecular architecture and the structural basis for anion interaction in prestin and SLC26 transporters. Nat. Commun. 5:3622 doi: 10.1038/ncomms4622 (2014).